Crystal structure of a plectonemic RNA supercoil Genome packaging is an essential housekeeping process in virtually all organisms for proper storage and maintenance of genetic information. Although the extent and mechanisms of packaging vary, the process involves the formation of nucleic-acid superstructures. Crystal structures of DNA coiled coils indicate that their geometries can vary according to sequence and/or the presence of stabilizers such as proteins or small molecules. However, such superstructures have not been revealed for RNA. Here we report the crystal structure of an RNA supercoil, which displays one level higher molecular organization than previously reported structures of DNA coiled coils. In the presence of an RNA-binding protein, two interlocking RNA coiled coils of double-stranded RNA, a 'coil of coiled coils', form a plectonemic supercoil. Molecular dynamics simulations suggest that protein–RNA interaction is required for the stability of the supercoiled RNA. This study provides structural insight into higher order packaging mechanisms of nucleic acids. Protein-mediated condensation of nucleic acids is an essential component of cellular mechanisms involving genetic regulation and storage. Whereas the smaller, circular plasmid DNA of prokaryotes prefers a plectonemic arrangement, the structure of eukaryotic chromatin, as observed in the nucleosome, adopts a solenoidal coil of DNA through histone mediation [1] , [2] . The structural similarities observed for helical forms of DNA and double-stranded (ds) RNA suggest that both nucleic acid types are capable of forming similar higher order structures. Although RNAs are not involved in the storage of genetic information in free-living organisms, both single-stranded (ss) and dsRNA viruses possess densely packaged RNA genomes. Electron microscopy studies have shown that dsRNA-virus genomes form supercoils within the virus particles [3] , [4] , [5] . Some ssRNA viruses demonstrate similar genome packaging through the formation of hairpin structures that are arranged into triangles and/or pentagons according to virion symmetry [6] , [7] , [8] , [9] . Thus, it is clear from these studies that RNA, like DNA, is capable of forming higher order structures that facilitate the protection, storage, and handling of genetic material. However, detailed structural information for higher order assemblies of RNA, as well as for supercoiled DNA, has been until now unavailable. The N utilization substance proteins B and E (NusB and NusE) interact with BoxA RNA during the initiation of transcription antitermination. To demonstrate how the NusB–NusE heterodimer recognizes a BoxA sequence, we previously determined the crystal structure of Aquifex aeolicus ( Aa ) NusB–NusE in complex with a ss12-mer BoxA RNA ( Aa NusB–NusE-BoxA, Protein Data Bank (PDB) accession code 3R2C ) [10] . At lower temperatures, however, this RNA self-hybridizes to form a duplex with 2-nucleotide (nt) 5′ overhangs ( Supplementary Fig. S1 ). Taking advantage of this phenomenon, we have also previously determined the crystal structure of Aa NusB–NusE in complex with dsRNA ( Aa NusB–NusE–dsRNA, PDB accession code 3R2D ) [10] , and in this present study, Aa NusB in complex with dsRNA ( Aa NusB–dsRNA). In the Aa NusB-NusE–dsRNA structure, the 12-mer dsRNA exists as a single duplex [10] , whereas in the Aa NusB–dsRNA structure, this duplex forms a pseudo-continuous double helix. Polymerization of small duplexes to form a pseudo-continuous double helix is common for both nucleic acid types. For example, a DNA pseudo-helix is formed by a 12-mer dsDNA with 2-nt 5′ overhangs (PDB accession code 1AF1 ) [11] , and an RNA pseudo-helix is formed by an 11-mer dsRNA with 2-nt 3′ overhangs (PDB accession code 2NUG ) [12] . The pseudo-continuous helices assume different forms in different structures. The aforementioned DNA pseudo-helix exists as coiled coils [11] , whereas the RNA pseudo-helix exists as straight A-form dsRNA [12] . Strikingly, the RNA pseudo-helix in the Aa NusB–dsRNA structure assumes the form of coiled coils, and two such coiled coils form a protein-stabilized RNA supercoil. Overall structure of Aa NusB-stabilized RNA supercoil Here we report the crystal structure of an Aa NuB-stabilized RNA supercoil at 3.2-Å resolution ( Fig. 1 ; Supplementary Table S1 ). The repeating unit of the RNA is the aforementioned ss12-mer RNA, which self-hybridizes to form a duplex with 2-nt 5′ overhangs ( Supplementary Fig. S1 ). The RNA duplexes noncovalently self-polymerize via these overhangs, giving rise to a pseudo-continuous double helix that approximates A′-form dsRNA. Each of these double helices interacts with another to form a plectoneme ( Supplementary Fig. S2 ), which is stabilized by Aa NusB protein in an RNA-sequence-independent manner ( Supplementary Fig. S3 ). The global structure in the crystal lattice exists as a continuous array of protein-mediated RNA supercoils, which are evenly spaced and run parallel to the c axis of the crystal lattice ( Fig. 1a ). 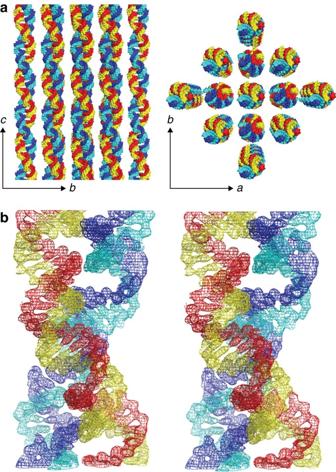Figure 1: Crystal structure of the plectonemic RNA supercoil. (a) The global structure exists as a continuous network of protein-mediated RNA supercoils, which are evenly spaced and run parallel to thecaxis of the crystal lattice. Unit cell directions are indicated, but the protein molecules are omitted for clarity. (b) Electron density (2Fo-Fcmap contoured at 1.0σ) in stereo for the two plectonemic RNA coiled coils, colour-coded by strand (coil 1: blue/cyan; coil 2: red/yellow). Figure 1: Crystal structure of the plectonemic RNA supercoil. ( a ) The global structure exists as a continuous network of protein-mediated RNA supercoils, which are evenly spaced and run parallel to the c axis of the crystal lattice. Unit cell directions are indicated, but the protein molecules are omitted for clarity. ( b ) Electron density (2 F o - F c map contoured at 1.0σ) in stereo for the two plectonemic RNA coiled coils, colour-coded by strand (coil 1: blue/cyan; coil 2: red/yellow). Full size image The crystal contains a solvent:protein:RNA volume ratio of 0.60:0.29:0.11. The asymmetric unit contains four copies of the Aa NusB dimer and a section of the RNA supercoil, 60 nt in length ( Supplementary Fig. S3 ). An apparent screw disorder exists along the axis of each coiled coil, a common crystallographic phenomenon observed among structures of nucleic acids [13] . Such screw-related disorder reflects the inherent variations in register of dsRNA with respect to bound protein molecules, which is consistent with the observation that all protein–RNA interactions are independent of nucleotide sequence. In addition, the higher order assembly of the synthetic 12-mer RNA, which lacks a 5′-terminal phosphate group, does not reveal the otherwise expected gaps in electron density within each pseudo-continuous strand—an ambiguity that is also evident among the most base pairs (bp) ( Fig. 1b ). The heterogeneity of the RNA register likely contributes to the moderately low resolution (3.2 Å) and high atomic displacement factors (89.9 Å 2 by average) of an otherwise well-ordered structure ( Supplementary Table S1 ). Aa NusB interacts with both minor and major grooves of RNA Each of the two subunits of the Aa NusB protein dimer uniquely interacts with the RNA supercoil. A-type Aa NusB molecules (chains A, C, E and G) interact with both the minor and major grooves of the RNA pseudo-helix ( Fig. 2 ), whereas the dsRNA interaction with B-type Aa NusB molecules (chains B, D, F and H) likely results from the dimerization of Aa NusB, and aids in crystal packing. In both cases, however, the buried surface areas are relatively small (860 Å 2 and 220 Å 2 for Aa NusB types A and B, respectively). 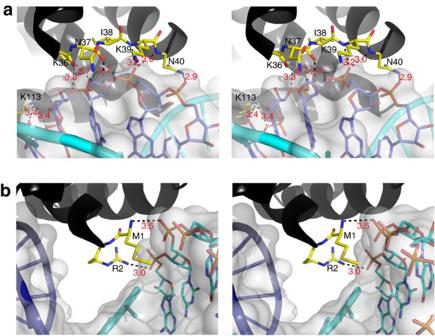Figure 2: Stereo representations of the interactions of A-typeAaNusB molecules with dsRNA. Residues ofAaNusB and RNA involved in direct protein–RNA interactions are shown as sticks, with hydrogen-bond distances reported in Å, shown in red. (a) Binding ofAaNusB to the minor groove of RNA. (b) Interaction between the N-terminus ofAaNusB and the major groove of RNA. Figure 2: Stereo representations of the interactions of A-type Aa NusB molecules with dsRNA. Residues of Aa NusB and RNA involved in direct protein–RNA interactions are shown as sticks, with hydrogen-bond distances reported in Å, shown in red. ( a ) Binding of Aa NusB to the minor groove of RNA. ( b ) Interaction between the N-terminus of Aa NusB and the major groove of RNA. Full size image The minor-groove-binding region of A-type Aa NusB is consistent with that observed in the Aa NusB-NusE–dsRNA structure (PDB accession code 3R2D ) [10] . Among 8 hydrogen bonds formed between five Aa NusB residues (K36, N37, K39, N40 and K113) and the backbone of dsRNA at the minor groove ( Fig. 2a ), only one (involving N40) is not seen in the Aa NusB-NusE–dsRNA structure ( Supplementary Fig. S4 ). Uniquely, however, the A-type Aa NusB molecule wedges its amino-terminal helix into the major groove of the RNA helix and secures such interaction with two hydrogen bonds ( Fig. 2b ). This protein-major groove interaction is not observed in the Aa NusB-NusE–dsRNA structure (PDB accession code 3R2D ) [10] owing to the limited size and absence of polymerization of the RNA duplex ( Supplementary Fig. S4 ). To test the role of protein–RNA interactions in the structural integrity and stability of the RNA supercoil, we have conducted molecular dynamics (MD) simulations for two systems based on the content of the asymmetric unit: four copies of the Aa NusB dimer and one section of the RNA supercoil ( Supplementary Fig. S3 ). System I contains the RNA supercoil only. MD simulation suggests that the RNA supercoil is unstable in the absence of protein, demonstrated by a steep rise in the root-mean-square deviation, relative to the crystal structure, to a value above 15 Å. System II, on the other hand, which contains the RNA supercoil bound by the eight Aa NusB molecules, shows a gradual change in the root-mean-square deviation, which plateaus at ~6 Å during the MD simulation ( Supplementary Fig. S5 ). These results indicate that the protein–RNA interactions are required for RNA-supercoil stability. The RNA supercoil features a widened major groove A systematic structural analysis was performed by measuring the helical parameters for each of the coiled coils comprising the crystallographic repeating unit of supercoiled RNA (coil 1: chains a–j, coil 2: chains k–t, Table 1 ). Given the moderately low resolution, presence of screw disorder, and suboptimal base pairing ( Supplementary Fig. S1 ), nonuniformity throughout the coiled coils is expected. However, when averaged, the helical parameters for each coiled coil of dsRNA are most consistent with the A′ conformation, which is emphasized by large major groove widths ( Table 1 ). The widening of the major groove is induced, at least in part, by the insertion of A-type Aa NusB molecules, in which the N-terminal amino group of the protein interacts with the RNA backbone ( Fig. 2b ). This observation is in agreement with previous findings, which indicated that the wider major groove of A′-RNA is more accommodating for interactions with proteins [14] . Also, the genetic material from a dsRNA virus was confirmed to be in the A′ configuration [15] , suggesting that protein-stabilized RNA supercoils may provide biological relevance with respect to dsRNA-virus genome packaging. Table 1 Helical parameters for RNA and DNA duplexes. Full size table As aforementioned, structures of other RNA coiled coils are not available. We therefore compared our structure with two structures of DNA coiled coils, PDB accession codes 2AF1 (ref. 11 ) and 1KX5 (ref. 16 ), as shown in Fig. 3 . Each structure was analysed by constructing a two-dimensional projection of the coiled coil(s) and measuring the diameter (width) and pitch (height) of one full turn of one coil, respectively ( Fig. 3a–c ). The most pronounced difference among these three structures is the plectonemic supercoiling of RNA, as opposed to the solenoidal architecture observed for the DNA coiled-coil structures. In the formation of the RNA supercoil ( Fig. 3d ), the tight braiding of coiled coils creates periodic helical kinks, leading to large deviations in major groove widths (9.4–15.6 Å). The minor grooves, on the other hand, show little variation (9.0–11.1 Å). In contrast, the continuous, nonuniform bending of the DNA superhelix in the structure of the nucleosome core particle (PDB accession code 1KX5 ) [16] reveals significant deviations in both major (8.9–15.6 Å) and minor (2.5–9.4 Å) groove widths ( Fig. 3f ); the 2.5-Å minor groove width is induced by the insertion of histone–arginine side-chains at several minor groove positions within the nucleosome DNA. In the absence of protein, however, the coiled-coiled DNA structure (PDB accession code 2AF1 ) [11] , formed by the d(CGATATATATAT) dodecamer, demonstrates only slight to moderate deviations for both major (13.7–14.3 Å) and minor (3.7–6.6 Å) groove widths ( Fig. 3e ). Together, the geometric variation among these superstructures reflects the degree of structural flexibility necessary for nucleic acids to achieve various functions and accommodate different molecular and cellular environments. 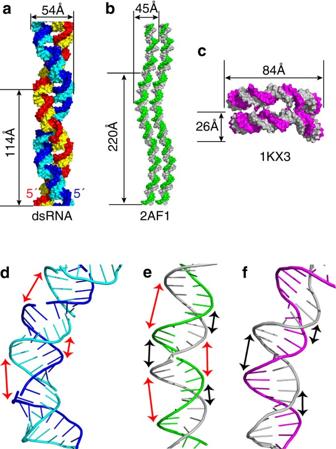Figure 3: Schematic illustrations of nucleic-acid superstructures. Shown are 1.5 or 2.0 turns of coiled coils, colour coded by individual strands, for crystal structures of (a) supercoiled RNA (this work), (b) coiled-coiled DNA (PDB accession code2AF1)11, and (c) nucleosome core particle DNA (PDB accession code1KX5)16. Pitch and diameter for each coil are indicated. The 5′ termini of the red strand of coil 1 and the blue strand of coil 2 of dsRNA are indicated in panela. Close-up view of the observed kinks in (d) supercoiled RNA, (e) coiled-coiled DNA, and (f) nucleosome core particle DNA, as illustrated by changes in major (in red) and minor (in black) groove widths. Figure 3: Schematic illustrations of nucleic-acid superstructures. Shown are 1.5 or 2.0 turns of coiled coils, colour coded by individual strands, for crystal structures of ( a ) supercoiled RNA (this work), ( b ) coiled-coiled DNA (PDB accession code 2AF1 ) [11] , and ( c ) nucleosome core particle DNA (PDB accession code 1KX5 ) [16] . Pitch and diameter for each coil are indicated. The 5′ termini of the red strand of coil 1 and the blue strand of coil 2 of dsRNA are indicated in panel a . Close-up view of the observed kinks in ( d ) supercoiled RNA, ( e ) coiled-coiled DNA, and ( f ) nucleosome core particle DNA, as illustrated by changes in major (in red) and minor (in black) groove widths. Full size image Further comparison of this structure of protein-associated RNA supercoils with previous studies of dsRNA-virus genomes indicates significant biological relevance. The supercoiled RNA in the crystal lattice has a nucleic-acid density of 42 bp per 100 nm 3 . Intriguingly, the average genome packing density of dsRNA viruses is ~40 bp per 100 nm 3 (refs 17 , 18 ). Furthermore, this RNA supercoil is left-handed. This feature is consistent with the left-handed helical filaments observed in untreated Moloney murine leukaemia virus, which were considered to be representative of the nucleocapsid [19] . Protein-coated plectonemic supercoils of the Drosophila X virus dsRNA genome also seem to be left-handed [15] . Given the diversity of dsRNA-binding proteins (dsRBPs), it is likely that other proteins of this type facilitate similar condensation and packaging mechanisms. It has been shown, for example, that a human dsRBP, Staufen, is selectively incorporated into virion particles of human immunodeficiency virus and other retroviruses by aiding in viral genome encapsidation and packaging, thus serving an important role in virion assembly and infectivity [20] . In summary, on comparison with higher order structures of both DNA and RNA, the structure of the RNA supercoil highlights the versatility of nucleic acids in high-density environments. These results not only increase our understanding of the coiled coiling and supercoiling phenomena of nucleic acids, but also provide a detailed model for the use of these superstructures in achieving essential cellular functions, such as gene regulation and genome packaging. Furthermore, the Aa NusB protein, given its sequence-independent interactions with supercoiled RNA, could potentially be utilized to promote the formation and/or crystallization of other nucleic-acid superstructures, or in the construction of novel nanostructures. Macromolecular crystallography The synthetic 12-mer RNA (5′-GGCUCCUUGGCA-3′) used in this experiment is the Aa BoxA RNA used in our previous work [10] . Aa NusB was cloned, expressed, and purified as described [21] with slight modifications. Briefly, The open reading frame encoding NusB (AAC06491) was amplified from genomic DNA by the PCR using the following oligodeoxyribonucleotide primers: (A) 5′-CCT CCG CAT ATG AGG TAT CGG AAAGGT GCA AG-3′ and (B) 5′-TCC CGC GGA TCC ATT ACT CTG ATT TTA AAC TTG GTT TTT CTT C-3′. The resulting PCR amplicon was cleaved with Nde I and Bam HI and then ligated with the NdeI/BamHI vector backbone of pET11c (Novagen, Madison, WI, USA) to create the Aa NusB expression vector pKM772. The nucleotide sequence of the insert was confirmed by DNA sequencing. pKM772 bearing BL21* (DE3) frozen stock cells were grown in 1 ml (LB with carbenicillin) at 37 °C for 6 h, followed by addition of 50 ml fresh media. The cells were incubated overnight at 37 °C. The overnight culture was added directly to 1 l fresh LBC media and allowed to grow at 37 °C. The protein was induced at an A600 nm=0.8–1.0, using 1 mM isopropylthiogalactoside and grown at 37 °C for 4 h after induction. Cells were collected by centrifugation. Cell pellet was re-suspended in 30 mM NaPO4 buffer at pH 6.8. Cells were cracked by sonication and heated to 90 °C for 30 min. The lysate was then centrifuged and the supernatant was applied to an SP sepharose ion-exchange column and eluted with 1 M NaCl in 30 mM NaPO4 buffer with a linear gradient. The purity of the protein was assessed by SDS–PAGE and/or by mass spectroscopy. Crystals of Aa NusB-RNA were grown at room temperature in 2-μl hanging drops containing equal volumes of protein solution (430 μM Aa NusB and 525 μM RNA in 25 mM Tris pH 7.5, 50 mM NaCl, and 1 mM EDTA) and well solution (0.2 M ammonium sulfate and 26% PEG-3350 in 0.1 M HEPES pH 7.5). A crystal of Aa NusB-RNA was soaked in a cryoprotectant solution containing 0.1 M HEPES pH 7.5, 0.2 M ammonium sulfate, 30% PEG-3350, and 5% glycerol, and flash-cooled in liquid nitrogen. X-ray diffraction data were collected at the Advanced Photon Source and processed with the HKL-3000 program suite [22] . Molecular replacement was performed using Phaser [23] . The Aa NusB-RNA structure was solved using the Aa NusB component in the Aa NusB-NusE–dsRNA structure (PDB accession code 3R2D ) [10] , as a search model. The structure was initially solved assuming tetragonal space group P4 1 2 1 2, but the symmetry was reinterpreted during refinement to be of the C2 monoclinic space group. Because of the specific coincidence of unit cell dimensions, the occurrence of crystal twinning was checked and ruled out. Model building and refinement were carried out using the COOT [24] and PHENIX [25] programs with non-crystallographic symmetry restraints applied during refinement. The RNA sequence was assigned based on the Aa NusB-NusE–dsRNA structure (PDB accession code 3R2D ) [10] . Because of the absence of 5′ phosphate groups, combined with the heterogeneity of RNA register, the 3′ and 5′ termini of adjacent strands of RNA were refined with a fixed distance of 2.5 Å as to reflect a continuous RNA helix. The final model was validated using MolProbity [26] . All figures were generated using PyMol [27] . Data collection and refinement statistics is summarized in Supplementary Table S1 . Molecular dynamics simulations MD simulations were performed using the NAMD package [28] and the Charmm 27 force field [29] , [30] , with constant pressure ensembles (NPT) at 1 atm and a temperature of 300 K. The time step was 2 fs with a SHAKE constraint on all bonds with hydrogen atoms. Productive MD runs were performed after 5,000 steps of minimizations and three 150 ps heating and equilibration runs. Long-range electrostatic interactions were calculated using the Particle Mesh Ewald method [31] . The starting conformations for both systems (System I and System II) were based on the crystal structure, and the missing amino-acid residues were added in random conformation. The simulated molecules were solvated in a TIP3P water box with a margin of at least 10 Å from any edge of the water box. To make the overall system neutral, the program Ionize (Theoretical and Computational Biophysics Group, University of Illinois at Urbana-Champaign, http://www.ks.uiuc.edu/Development/MDTools/ionize/license.html ) was used to place sodium ions around the negatively charged regions of the RNA. Additional sodium and chloride ions were added to each system to reach an ionic concentration of 0.25 M. Acccession codes: The structural coordinates and diffraction data of Aa NusB-RNA have been deposited in the Protein Data Bank under accession code 4EYA . How to cite this article: Stagno, J. R. et al . Crystal structure of a plectonemic RNA supercoil. Nat. Commun. 3:901 doi: 10.1038/ncomms1903 (2012).